Bridging quantum and classical plasmonics with a quantum-corrected model Electromagnetic coupling between plasmonic resonances in metallic nanoparticles allows for engineering of the optical response and generation of strong localized near-fields. Classical electrodynamics fails to describe this coupling across sub-nanometer gaps, where quantum effects become important owing to non-local screening and the spill-out of electrons. However, full quantum simulations are not presently feasible for realistically sized systems. Here we present a novel approach, the quantum-corrected model (QCM), that incorporates quantum-mechanical effects within a classical electrodynamic framework. The QCM approach models the junction between adjacent nanoparticles by means of a local dielectric response that includes electron tunnelling and tunnelling resistivity at the gap and can be integrated within a classical electrodynamical description of large and complex structures. The QCM predicts optical properties in excellent agreement with fully quantum mechanical calculations for small interacting systems, opening a new venue for addressing quantum effects in realistic plasmonic systems. The capability of plasmonic systems to control, localize and enhance optical signals at the sub-wavelength scale has paved the way for many novel concepts and applications in nanophotonics [1] , [2] , [3] , [4] , [5] , [6] , [7] , [8] , [9] , [10] . The tremendous progress in experimental techniques and fabrication of nano-plasmonic devices has stimulated theoretical development for addressing complex physical phenomena occurring at sub-nanometric scale. Presently, most theoretical descriptions of the optical response of plasmonic systems rely on classical electromagnetic models (CEM) describing the response of the structures by a frequency-dependent local linear dielectric function that characterizes each individual part of the nanostructure. In this classical approach, the interface between the different materials is assumed abrupt, and quantum-mechanical effects due to the electron density spill-out from the nanoparticles and interparticle electron tunnelling are not considered. While the classical approach has been successfully used to calculate the optical properties of many different plasmonic systems, special care must be taken when the separation distances involved are at the nanometre or sub-nanometre scale [11] , [12] . In this situation, solving Maxwell equations using non-local bulk dielectric functions ( k , ω ) (refs 13 , 14 , 15 , 16 ) may extend the validity of the classical treatment. However, this approach cannot describe properly the electron tunnelling for small separations when the electronic densities of the individual nanostructures overlap. In such a case, a quantum-mechanical approach that fully accounts for non-local effects is necessary [17] . One example of such a quantum model (QM) is the time-dependent density functional theory (TDDFT) [18] , [19] that offers a possibility to address the optical response of plasmonic systems at the fully quantum ab initio level. Recent studies have demonstrated that the tunnelling current between nanoparticles shortcircuits the junction, reduces the Coulomb coupling between charges of opposite sign in the two nanoparticles and strongly affects the optical response of the system [20] , [21] , [22] . In general, quantum effects can completely change the spectral distribution and the field enhancements of the resonant modes supported by a given plasmonic structure, thus limiting the validity of a classical description. Consideration of such quantum effects is therefore of paramount importance in systems with sub-nanometer wide gaps, which nowadays gain a lot of interest owing to their importance as substrates in plasmon-enhanced spectroscopies such as surface-enhanced Raman scattering [12] , [23] or in the optoelectronic response of hybrid systems [9] . The signal intensity of such spectroscopies depends on the local electromagnetic field enhancement [24] , [25] , [26] and can be strongly reduced when electron transfer sets in across the junction. A quantum treatment of the optical properties of large plasmonic systems is very demanding, owing to the high number of electrons involved in the optical response. Thus, previous studies of nanoparticle dimers using fully quantum-mechanical models were limited to small spheres [20] , [21] with a few thousand conduction electrons. In contrast, typical plasmonic systems used in experiments contain many millions or even billions of electrons and cannot be currently addressed with first-principle methods. In this article, we introduce a method to study the optical response of large coupled plasmonic systems that includes quantum effects. In this approach, which we denote the quantum-corrected model (QCM), the junction between two adjacent nanoparticles is represented with a fictitious conductive material that mimics the electron tunnelling. With the inclusion of this medium, the optical properties can be calculated within a classical electrodynamic framework [27] and yield excellent agreement with fully quantum-mechanical calculations for small spheres. By applying the QCM introduced here, we observe quantum-induced effects in sub-nanometer gaps of large metallic dimers and bowtie antennas, such as spectral redistribution of electromagnetic modes and collapse of the field enhancement. 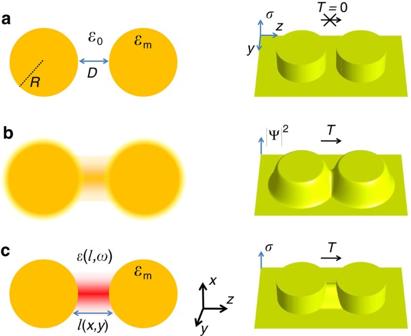Figure 1: Description of the material properties of a metallic dimer within the classical and quantum treatments. Schematics of a metallic dimer composed of two spherical particles separated by a distanceDwith use of a (a) CEM, (b) QM and (c) QCM. The schematics show the variation of the dielectric properties of the materials at the boundaries of the dimers. The joint sketches show the corresponding absolute value of the conductivityσ(a,c) and electron density distribution |Ψ|2(b). Within a classical framework (a), the conductivity is different from zero only inside the spheres and no electron transfer can occur between the particles (electron tunnelling probabilityT=0). In a fully quantum-mechanical treatment (b), the density of electrons in the gap is non-zero for smallDand tunnelling is possible (T>0). In the QCM (c), the electron tunnelling is accounted for by describing the material in the junction with a fictitious dielectric medium (illustrated by a shaded red colour) characterized by a local dielectric permitivity(l(x,y),ω) that depends only on the local widthl(x,y) of the junction and the nanoparticle material at both sides. Quantum-corrected model Figure 1 illustrates the idea underlying the QCM for the case of two metallic spheres of radius R surrounded by vacuum with permitivity 0 and separated by a distance D . Within the classical description, the interface between the different materials is assumed abrupt, as sketched in Fig. 1a . In the simplest approach, a Drude model characterized by a bulk plasma frequency ω p and damping parameter γ p can describe the dielectric response of a metal as Figure 1: Description of the material properties of a metallic dimer within the classical and quantum treatments. Schematics of a metallic dimer composed of two spherical particles separated by a distance D with use of a ( a ) CEM, ( b ) QM and ( c ) QCM. The schematics show the variation of the dielectric properties of the materials at the boundaries of the dimers. The joint sketches show the corresponding absolute value of the conductivity σ ( a , c ) and electron density distribution |Ψ| 2 ( b ). Within a classical framework ( a ), the conductivity is different from zero only inside the spheres and no electron transfer can occur between the particles (electron tunnelling probability T =0). In a fully quantum-mechanical treatment ( b ), the density of electrons in the gap is non-zero for small D and tunnelling is possible ( T >0). In the QCM ( c ), the electron tunnelling is accounted for by describing the material in the junction with a fictitious dielectric medium (illustrated by a shaded red colour) characterized by a local dielectric permitivity ( l ( x , y ), ω ) that depends only on the local width l ( x , y ) of the junction and the nanoparticle material at both sides. Full size image The parameter ∞ describes the dielectric screening introduced by the bound valence electrons of the positive ion cores and the second term is the contribution from the conduction electrons. In what follows we will for simplicity assume ∞ =1. The schematic in Fig. 1a represents the dielectric permitivity in the different parts of the metallic dimer together with the corresponding local conductivity σ =− iω ( −1)/(4 π ), which is given by the electronic density distribution and is zero in vacuum. In this classical formalism, zero conductivity in the junction implies that the probability of electron tunnelling T between the nanoparticles is zero. In a QM, however, there is no abrupt change of the electron density at the interfaces of the nanoparticles, as represented in Fig. 1b . The density of electrons |Ψ| 2 varies continuously between the metal surfaces in this case, and can be significant in the centre of the junction for narrow gaps. This overlap of the evanescent electron densities for small separation distances (subnanometric) sets in the possibility of electron tunnelling between the two spheres. The smaller the interparticle separation is, the larger the electron tunnelling probability. Figure 1c introduces the QCM schematically. Outside the gap region, the particle and the surrounding vacuum are described by the conventional dielectric permittivities with abrupt interfaces. We use the same Drude metal model as in equation (1), with fixed plasma frequency ω p and damping parameter γ p to describe the material of both particles. The red-shaded region at the gap in Fig. 1c represents the fictitious material that will account for electron tunnelling. It is possible to build the local permittivity ( l , ω ) corresponding to this fictitious material as a function that depends on the separation distance between interfaces l , for each lateral position in the gap l = l ( x , y ). This permittivity ( l , ω ) can be obtained from a quantum-mechanical calculation of the electron transmission probability T ( l ) through the potential barrier separating the two metals, as will be described below. In order to obtain ( l , ω ), we consider now the relationship between the conductivity σ( l , ω ) and the dielectric function (in atomic units) and assume a Drude model to characterize the local permittivity of the fictitious medium at the gap, where the plasmon frequency of the fictitious material ω g and the screening contribution ∞ are assumed to be equal to that of the surrounding material ( ω g =ω p , ∞ =1), and the tunnelling damping γ g ( l ) is a function of the separation distance l ( x , y ) at the particular lateral position of the gap ( x , y ). The separation-dependent tunnelling damping γ g ( l ) is thus the key parameter describing the quantum tunnelling resistance introduced by the presence of the gap. We can obtain γ g ( l ) from the static conductivity σ 0 ( l )= σ ( l , ω →0), yielding: This procedure can be generalized to situations with ∞ ≠1, that is, where screening due to bound electrons would be present. In our model, we assume a value of ω g = ω p and consider γ g as the varying parameter because, as will be discussed below, this choice is consistent with the resistive nature of the gaps found in the full-quantum-mechanical calculations with TDDFT. Indeed, as γ g ω over a broad range of interparticle separations, the frequency dispersion of the conductivity is negligible and thus σ ( l , ω ) can be determined by the dc value σ 0 . This large tunnelling resistance makes the results of the plasmonic response unsensitive to the specific parameterization of the permittivity of the fictitious medium as long as it properly accounts for the resistive character of the gap. The robustness of the model to different choices of parametrization of ω g and γ g is explicitly illustrated in the Supplementary Fig. S1 and in the Supplementary Discussion . Tunnelling probability and conductivity in the SSTM approach To obtain the conductivity as a function of separation distance l , we need to relate the current J and the field E in the junction. To do so, we note that the electric field E in the junction is predominantly oriented along the interparticle axis, and it is nearly independent of the z coordinate. Moreover, the transmission of electrons at the Fermi energy, Ω F (which are the electrons that will dominate the tunnelling current) through the potential barrier separating the nanoparticles occurs at a time scale much smaller than the optical cycle for sufficiently large separation distances l . Thus, the tunnelling current adiabatically follows the field in the junction. Under these assumptions, a dc or static scanning tunnelling microscopy (SSTM) approach can be used. For the typical sizes of plasmonic nanoparticles, the radii of curvature of the surfaces are much larger than both the Fermi electron wavelength and the typical separation distances at which quantum effects become important. The tunnelling current density in a given portion of the gap ( x , y ) with separation l ( x , y ) can thus be approximated by the current density obtained in a simpler system, as that of the two flat metal surfaces represented in Fig. 2a , separated by the same distance l . 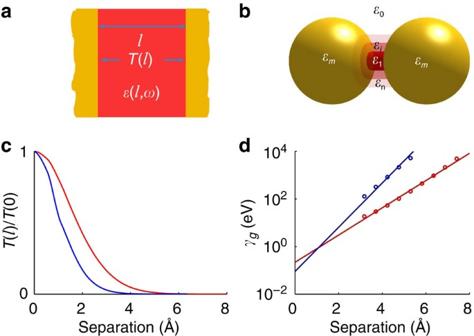Figure 2: Geometries and parameters involved in the QCM. (a) Simpler plasmonic system composed of two semi-infinite planar interfaces separated by a distanceland characterized by tunnelling transmissionT(l). The tunnelling-induced conductivity between the surfaces defines the separation-dependent dielectric material(l,ω) used in the QCM. (b) Schematics indicating the inhomogeneous distribution of the local dielectric constant used in the QCM in the case of the metallic dimer.mis the dielectric constant of the metal,0the vacuum permittivity andithe separation-dependent dielectric constant of the shells of fictitious material that accounts for the quantum tunnelling (i=1,...,n). In the figure, three of these representative concentric shells are shown within the gap. (c) Normalized electron tunnelling transmissionT(l)/T(0) and (d) tunnelling dampingγgas a function of separation distancel. The open points in (d) correspond to values obtained from the SSTM approach. The full lines in (d) correspond to the values used in the model exponential approach adopted in the QCM. In both (c) and (d), red corresponds to the Na jellium material and blue to the Au jellium. Figure 2: Geometries and parameters involved in the QCM. ( a ) Simpler plasmonic system composed of two semi-infinite planar interfaces separated by a distance l and characterized by tunnelling transmission T ( l ). The tunnelling-induced conductivity between the surfaces defines the separation-dependent dielectric material ( l , ω ) used in the QCM. ( b ) Schematics indicating the inhomogeneous distribution of the local dielectric constant used in the QCM in the case of the metallic dimer. m is the dielectric constant of the metal, 0 the vacuum permittivity and i the separation-dependent dielectric constant of the shells of fictitious material that accounts for the quantum tunnelling ( i =1,..., n ). In the figure, three of these representative concentric shells are shown within the gap. ( c ) Normalized electron tunnelling transmission T ( l )/ T (0) and ( d ) tunnelling damping γ g as a function of separation distance l . The open points in ( d ) correspond to values obtained from the SSTM approach. The full lines in ( d ) correspond to the values used in the model exponential approach adopted in the QCM. In both ( c ) and ( d ), red corresponds to the Na jellium material and blue to the Au jellium. Full size image Within the SSTM approach, the distance-dependent dc conductivity σ 0 ( l ) at the junction under bias U = lE can be connected with the current density J following [28] where T (Ω, l ) is the energy Ω-dependent electron tunnelling probability at each lateral position within the gap with separation l . This transmission probability can be obtained within a fully quantum-mechanical treatment as the number of electrons to treat in such a system (simple flat gap) is relatively small. The quantum calculation of T (Ω, l ) can be tackled either from full ab initio approaches, accounting for atomistic structure or from a model potential approach. We use the second strategy for simplicity and assume tunnelling between jellium-like surfaces. More general and precise quantum-mechanical treatments based on atomistic models and Green's function techniques [29] can also be implemented to obtain the dc conductivity σ 0 ( l ). The QCM approach thus amounts to replacing the dielectric function at each lateral position ( x , y ) of the junction between the two nanoparticles ( Figs 1c and 2b ) by that obtained from a simpler situation ( Fig. 2a ) following equations (3), (4), (5). In Fig. 2c,d we represent the normalized values of the tunnelling transmission corresponding to the simplified system in Fig. 2a and its corresponding tunnelling damping γ g ( l ) as obtained from equations (4) and (5) for two metallic materials: Na and Au. The results of γ g ( l ) within the SSTM approach are shown only for intermediate and large separations in Fig. 2d , as the SSTM approach to the tunnelling current calculation is only valid in the regime where the transmission T is small. Noting that the calculated values of γ g ( l ) follow quite closely an exponential dependence with separation distance l (a well-established law for tunnelling processes), we assume for simplicity that this functional form is valid over the whole range of separations. The exponential expression describing γ g ( l ) is determined from the value at contact ( l →0) together with the SSTM results at large l . First, we impose that the tunnelling damping for zero gap distance γ g (0) is given by the value of the intrinsic damping of the metals at both sides of the cavity γ p , that is, γ g (0)= γ g ( l →0)= γ p , so that a continuous metal is formed. Furthermore, we choose that our exponential expression reproduces the SSTM results for a separation distance l ′ that gives a transmission coefficient T ( l ′)=0.01. The corresponding value of γ g ( l ) is shown as solid lines in Fig. 2d for Na and Au, demonstrating that the exponential approximation reproduces well the SSTM results for l 3 Å. We show in Supplementary Fig. S1 and in the Supplementary Discussion that the QCM is very robust with respect to the choice of particular distance l ′ and thus of T ( l ′). The calculation of γ g ( l ) from σ 0 ( l ), according to equation (4), allows to obtain ( l , ω ) by applying equation (3). However, the permittivity ( l , ω ) in a gap between nanoparticles is in general inhomogeneous. This inhomogeneity is accounted for within our QCM implementation by describing the gap region by a finite number n of regions with homogeneous permittivity i = ( l i , ω ), as sketched in Fig. 2b in the case of a dimer. Details of the implementation of the QCM within a classical electrodynamical calculations are given in the Methods. QCM versus QM in a small plasmonic dimer To examine the validity of our method, we compare in Fig. 3 the optical extinction and local field enhancement spectra obtained from a fully QM and from the QCM for a nanoparticle dimer consisting of two small metallic spheres of radius R with the incident electric field E 0 polarized along the dimer axis z . The QM calculations are performed using the TDDFT approach [30] with the nanospheres described within a spherical jellium model (JM). The simplicity introduced by the JM allows a sufficiently large number of valence electrons to be included within each nanosphere ( N e =1,074) so that the plasmonic modes are well developed [31] . Within the JM, the ionic cores of the atoms are represented with a uniform background charge density confined within the sphere of radius R . In the JM, the surface (jellium edge) is located at half a lattice spacing (0.2–0.3 nm) outside the physical surface. We consider Na spheres that are separated by a distance D (shortest separation within the junction, which in the QM refers to distances between the jellium edges of each surface). We also treat slightly overlapping situations ( D <0). The properties of a material in the JM are characterized by the Wigner–Seitz radius r s . The Na metal is taken here as a prototype system for the jellium description with r s =4 a.u. (1 a.u.=1 atomic unit ~0.529 Å) in the quantum calculations. In the Drude description of the QCM, we use ∞ =1, ω p =5.16 eV and γ p =0.218 eV. This choice ensures a proper correspondence between material properties in both models. 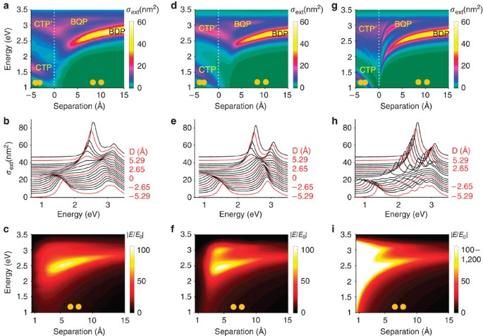Figure 3: Optical response of a small metallic dimer within quantum and classical models. Comparison of the optical properties of a metallic dimer obtained with (a–c) the full-QM, (d–f) with the QCM and (g–i) with a clasical electromagnetic model (CEM).The dimer consists of two Na spheres of radiusR~2.17 nm (40.96 a.u.) in vacuum, separated by a distanceD. The incoming field is a plane wave with electric fieldE0polarized along the dimer axisz. The centre of the particles are atz=±(R+D/2), andDis negative for overlapping spheres.D=−2Rwould correspond to the limit of a single sphere. (a,d,g) show colour plots of the extinction spectraσextof the dimers (far-field) as a function of separation distanceD.Dis expressed in Ångströms, and the extinction cross-section in nm2. Zero-separation distance is marked as a vertical dashed line separating the classical non-touching regime and the overlapping regime. Each of these regimes is schematically represented by separated and overlapping yellow dots, respectively. The most relevant modes are identified within the three treatments followed: bonding dimer plasmon (BDP), bonding quadrupolar plasmon (BQP), charge transfer plasmon (CTP) and higher-order charge transfer plasmon (CTP′). (b,e,h) Far-field spectra from selected distances in (a), (d) and (g), respectively. For clarity, a vertical shift proportional to the separation distance is used. Traces in red correspond to separation distances ofD=−5.29, −2.65, 0, 2.65 and 5.29 Å, as indicated on each graph. (c,f,i) Colour plots of the local field enhancement |E/E0| (near-field) at the centre of the junction for separationsD>0.5Å. The yellow dots schematically represent the particles in the non-touching regime. Figure 3: Optical response of a small metallic dimer within quantum and classical models. Comparison of the optical properties of a metallic dimer obtained with ( a–c ) the full-QM, ( d–f ) with the QCM and ( g–i ) with a clasical electromagnetic model (CEM).The dimer consists of two Na spheres of radius R ~2.17 nm (40.96 a.u.) in vacuum, separated by a distance D . The incoming field is a plane wave with electric field E 0 polarized along the dimer axis z . The centre of the particles are at z =±( R + D /2), and D is negative for overlapping spheres. D =−2 R would correspond to the limit of a single sphere. ( a , d , g ) show colour plots of the extinction spectra σ ext of the dimers (far-field) as a function of separation distance D . D is expressed in Ångströms, and the extinction cross-section in nm 2 . Zero-separation distance is marked as a vertical dashed line separating the classical non-touching regime and the overlapping regime. Each of these regimes is schematically represented by separated and overlapping yellow dots, respectively. The most relevant modes are identified within the three treatments followed: bonding dimer plasmon (BDP), bonding quadrupolar plasmon (BQP), charge transfer plasmon (CTP) and higher-order charge transfer plasmon (CTP′). ( b , e , h ) Far-field spectra from selected distances in ( a ), ( d ) and ( g ), respectively. For clarity, a vertical shift proportional to the separation distance is used. Traces in red correspond to separation distances of D =−5.29, −2.65, 0, 2.65 and 5.29 Å, as indicated on each graph. ( c , f , i ) Colour plots of the local field enhancement | E / E 0 | (near-field) at the centre of the junction for separations D>0.5 Å. The yellow dots schematically represent the particles in the non-touching regime. Full size image We first describe the results obtained within the full-QM in Fig. 3a–c . Analysing the extinction cross-section ( σ ext , far field) and local field enhancement (| E / E 0 |, near-field) in the centre of the junction, it is possible to distinguish three regimes showing different behaviour as a function of junction width D , which we denote as non-contact, tunnelling and contact regimes. In the non-contact regime, for distances D 5 Å, no significant electron transfer can occur between the nanoparticles and thus this situation can be correctly described within the classical electrodynamical treatment [2] , [32] , [33] , as shown in Fig. 3g–i . The dominant, lowest-energy bonding dipolar plasmon and the bonding quadrupolar plasmon at larger energy redshift as the separation distance becomes smaller. In this regime, the value at resonance of the local field enhancement increases monotonically as the spheres approach each other. In Fig. 3 and in the following figures, we report field enhancements in the centre of the junction. The actual location of the largest local field enhancement depends slightly on dimer separation but the quenching found relative to larger separation distances is independent of the evaluation point at the gap. In the contact regime characterized by a separation of D 1 Å, the conductance of the junction is large and the dimer behaves as a single non-spherical metallic structure. As the overlap increases, the modes blueshift towards the values of a single sphere. These modes are charge transfer plasmons (CTPs) characterized by an oscillatory current established between the two spheres [3] , [34] . The lowest-energy CTP resonance is at ≈1.5 eV, considerably lower energy than the modes in the non-contact regime. The excitation of CTP modes that blueshift for increasing overlap is also found within a classical treatment [3] , [35] , [36] ( Fig. 3g ), but quantum effects considerably modify both the width and spectral position of the modes. The tunnelling regime that lies in-between the contact and non-contact situations (1 Å D 5 Å) is of special interest in field-enhanced applications as the field enhancements in narrow plasmonic gaps are commonly expected to be large. This regime, which cannot be correctly modelled using a classical approach, is characterized by intermediate values of the tunnelling current through the junction. The electron transfer neutralizes the high charge densities on the opposite sides of the junction. As a result, the local field enhancement obtained within the QM for D 4 Å ( Fig. 3c ) shows a considerable decrease in magnitude [14] , [16] , [20] when compared with that obtained from CEM ( Fig. 3i ). Furthermore, the extinction cross-section in the QM shows a continuous and progressive transition between the modes of the contact and non-contact regimes ( Fig. 3a ), a feature totally missing in the CEM ( Fig. 3g ). The results from the QCM ( Fig. 3d–f ) successfully reproduce the optical spectra and near-field obtained using the QM in all three separation distance regimes. Notably, the QCM accurately describes the mode transition between the contact and non-contact regimes and the sharp decrease of local field enhancement for D ~4 Å. To facilitate the comparison and make it more quantitative, in Fig. 3b,e,h we show particular extracts of the extinction spectra at different separation distances as calculated with the QM, QCM and CEM. Apart from subtle differences, the overall quantitative agreement between the results obtained with QCM and those from full TDDFT calculations is excellent. Quantum plasmonics in large metallic systems Metallic particles in plasmonic applications are typically much larger than those considered in Fig. 3. The QCM introduced here offers the possibility to include quantum effects in the optical response of large-sized nanostructures. As an illustration of the power of the method, we now consider a dimer formed by two Au spheres of radius R =25 nm. To characterize the material response of Au, a value of ∞ =1, ω p =7.9 eV and γ p =0.09 eV are used in equation (1). This description does not account for the interband transitions that becomes important above 2.0 eV, but provides a good description of Au for large wavelengths. Before discussing the QCM results, and to better examine the shortcomings of the classical description, we first discuss the results obtained from the CEM. The extinction cross-section (far field) and the local field enhancement at the centre of the gap (near field) shown in Fig. 4a,b follow the trends obtained in Fig. 3g–i , as well as in similar systems treated classically [2] , [3] , [35] . As the two particle surfaces approach each other and charge concentrates at the metal interfaces in the gap region, the Coulomb interaction between the charge densities causes a significant redshift of the different modes. The local field enhancement associated with these resonances increases with decreasing distance [37] and can reach extremely high values. There is a sharp transition between the non-contact D >0 and the contact D <0 situations. Upon conductive contact, the modes acquire a CTP nature and blueshift as the overlap of the spheres increases. The large density of modes after contact is due to the presence of very sharp edges in the junction area resulting from the abrupt termination of the nanoparticle surfaces [38] , [39] , [40] . 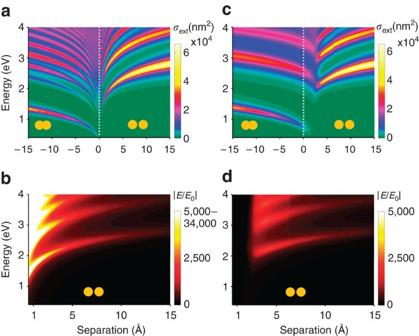Figure 4: Optical response of a large metallic dimer in a classical and quantum-corrected treatments. Comparison of the optical properties of a large plasmonic dimer treated (a,b) classically (CEM) and (c,d) within the QCM for different separation distancesD. The metallic spheres, with radiusR=25 nm, are described using Drude model parameters appropriate for jellium Au at large wavelengths∞=1,ωp=7.9 eV andγp=0.09 eV. The incoming field is a plane wave with electric fieldE0polarized along the dimer axis. The extinction cross-sectionσext(far-field) is represented in (a,c) and the local field enhancement at the central point between the spheres (near-field) is represented in (b,d) for separationD>0.5 Å. All distances are given in Ångströms, and the cross-section is expressed in nm2. Zero-separation distance is marked with a vertical dashed line in both (a) and (c). The non-touching regime is depicted schematically by two separated yellow dots, whereas the touching regime (negative separation distance) is depicted by two overlapping dots. Figure 4: Optical response of a large metallic dimer in a classical and quantum-corrected treatments. Comparison of the optical properties of a large plasmonic dimer treated ( a,b ) classically (CEM) and ( c,d ) within the QCM for different separation distances D . The metallic spheres, with radius R =25 nm, are described using Drude model parameters appropriate for jellium Au at large wavelengths ∞ =1, ω p =7.9 eV and γ p =0.09 eV. The incoming field is a plane wave with electric field E 0 polarized along the dimer axis. The extinction cross-section σ ext (far-field) is represented in ( a , c ) and the local field enhancement at the central point between the spheres (near-field) is represented in ( b , d ) for separation D >0.5 Å. All distances are given in Ångströms, and the cross-section is expressed in nm 2 . Zero-separation distance is marked with a vertical dashed line in both ( a ) and ( c ). The non-touching regime is depicted schematically by two separated yellow dots, whereas the touching regime (negative separation distance) is depicted by two overlapping dots. Full size image The QCM results for these large particles are shown in Fig. 4c,d for the extinction cross-section and field enhancement. As for the small dimer in Fig. 3 , it is possible to distinguish the contact, tunnelling and non-contact regimes. The non-contact regime extends down to somewhat smaller distances ( D 4 Å.) than for the smaller Na spheres. This is due to the higher work function of gold compared with that of Na, and therefore smaller electron tunnelling probability (see Fig. 2c ). Only in this non-contact regime, where tunnelling is negligible, do the QCM results resemble the classical results from the CEM. For separation distances below D ~4 Å the differences between CEM and QCM are striking. In the QCM contact regime D 1 Å, there are fewer modes, smaller blueshifts and often significantly enhanced broadening. The modes are excited already for small positive separation distances owing to the possibility of electron tunnelling. The transition from non-contact to contact regime is not sharp as in CEM, but progressive. While the CEM calculation shows a large number of modes, the QCM calculation only shows three distinct modes: a narrow CTP mode at low energy and two broader CTP modes at larger energies. Only the lowest-energy CTP mode has a direct correspondence with the CEM result and, as in Fig. 3 , it appears at energies considerably lower than the modes in the non-contact QCM regime. For the higher-order modes, the smoother edges of the junction area effectively spread out the induced charge density distribution and thus reduce the number of modes. We attribute the broadening of the CTP modes to dissipation associated with the electron current across the high resistance regions at the exterior of the junction. Another striking difference between the results obtained with the CEM and the QCM involves the collapse of the local field enhancement at resonance in the QCM with respect to the CEM. This collapse occurs at distances smaller than ~3.0 Å, that is, in the tunnelling regime. The fields are strongly suppressed near contact ( Fig. 4d ). In contrast, the CEM result in Fig. 4b shows a divergence of the enhancement up to contact. Similar results are obtained when the enhancement is evaluated at other optimal points of the central plane between the particles. The QCM thus opens a venue to estimate the suppression of the field enhancements in narrow junctions of large metallic structures, which is an important effect that needs to be considered when designing dimer junctions for field-enhanced applications. To further emphasize the importance of quantum effects in realistic nanostructures, we consider a gold bowtie antenna [7] , [41] , [42] , [43] as an example of a relevant plasmonic antenna [4] , [44] currently used in many plasmonic applications [6] . We model the bowtie antenna as two Au conical structures, 100 nm long and terminated near the gap with a spherical tips of 25 nm radius. 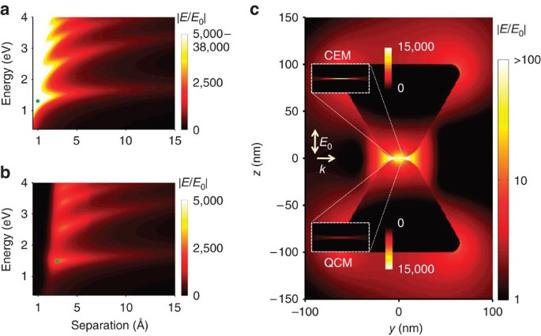Figure 5: Local electric field enhancement in a bowtie antenna using CEM and QCM. The nanoantenna is composed of two 100-nm-long cones in vacuum with a 25 nm radius spherical termination near the gap. The termination at the far-side from the gap is flat, with radius of curvature of 10 nm at the edges. The metal is described by a Drude dielectric function appropriate for jellium Au at large wavelengths, with∞=1,ωp=7.9 eV andγp=0.09 eV, and the structure is rotationally symmetric. The incident light is a plane wave polarized along the bowtie axis. (a) CEM and (b) QCM calculations of the local field enhancement as a function of separation distanceDat the central point in the gap. (c) Local field enhancement from QCM, with the insets showing a close up in a 4×2 nm2area including the gap for CEM, wavelengthλ=950 nm and separationD=1 Å, and QCM,λ=835 nm and separationD=3 Å. The corresponding positions are marked by green dots in panels (a,b). Notice that a logarithmic colour scale is used for the full structure, and a linear contour scale is used in the insets. Figure 5a,b shows the local field enhancement at the centre of the gap. The classical electrodynamic calculation ( Fig. 5a ) predicts very large (~38,000) and unphysical field enhancements for sub-nanometric separation D =0.5 Å. However, the QCM model predicts a much weaker enhancement ( Fig. 5b ), with a maximum of 3,000 at the optimal D~3 Å separation. Figure 5: Local electric field enhancement in a bowtie antenna using CEM and QCM. The nanoantenna is composed of two 100-nm-long cones in vacuum with a 25 nm radius spherical termination near the gap. The termination at the far-side from the gap is flat, with radius of curvature of 10 nm at the edges. The metal is described by a Drude dielectric function appropriate for jellium Au at large wavelengths, with ∞ =1, ω p =7.9 eV and γ p =0.09 eV, and the structure is rotationally symmetric. The incident light is a plane wave polarized along the bowtie axis. ( a ) CEM and ( b ) QCM calculations of the local field enhancement as a function of separation distance D at the central point in the gap. ( c ) Local field enhancement from QCM, with the insets showing a close up in a 4×2 nm 2 area including the gap for CEM, wavelength λ =950 nm and separation D =1 Å, and QCM, λ =835 nm and separation D =3 Å. The corresponding positions are marked by green dots in panels ( a , b ). Notice that a logarithmic colour scale is used for the full structure, and a linear contour scale is used in the insets. Full size image The spatial maps of the near-field distribution at the gap region in Fig. 5c illustrate this substantial difference. The insets show the fields in the gap area for resonant excitation for separation D =1 Å for classical electrodynamic calculations, and D =3 Å for QCM calculations. The wavelength and distance for the QCM inset correspond approximately to the optimum field enhancement, but the fields are still considerably weaker than those values obtained for the CEM. Quantum effects thus have a crucial role in reducing the plasmon-induced field enhancements and needs to be included when designing the structural parameters of the antenna. This finding stresses the importance of including quantum effects in any situation with closely spaced nanoparticles in plasmonic applications. In summary, we have proposed a straightforward method to incorporate quantum-mechanical effects within classical electromagnetic simulations of the optical properties of metallic nanostructures. With this general method, we have identified and quantified quantum effects determining the optical response of large metallic nanostructures with narrow gap junctions and slight overlap. The novel QCM approach can be applied generally to metallic nanostructures of arbitrary shape and size. The validity of the method has been corroborated for small systems by comparing their calculated optical properties with fully quantum-mechanical results. Different experimental techniques such as electromigration in gaps [23] , nanoscale positioning in scanning near-field optical microscopy [5] and light emission in scanning tunnelling microscopy [45] allow for exquisite control of sub-nanometer distances. These techniques show the potential to perform simultaneous optical characterization and transport measurements between metallic objects, opening the possibility to access the quantum effects discussed in this communication. The QCM approach thus provides the possibility to account for quantum effects in a variety of situations of relevance in nanophotonic applications, establishing a novel framework to address transport and optical properties in tunnelling configurations, as well as to tackle quantum effects in biochemical sensing and in molecular spectroscopy involving sub-nanometer scale photonics. Quantum-mechanical calculations within TDDFT To perform the fully quantum-mechanical calculations of the linear response of the plasmonic dimer and the time evolution of the electron densities and currents induced by the external laser pulse incident at the system, we use the Kohn–Sham (KS) scheme within TDDFT. The TDDFT is a state-of-the-art ab initio approach for the treatment of both the linear and nonlinear response to optical excitations in molecules and clusters [18] , [19] . The nanospheres are treated within the spherical JM allowing for modelling of a large number of conduction electrons so that the plasmonic modes are well developed. The ionic cores of the nanosphere atoms are represented by uniform background charge density (we use atomic units a 0 unless otherwise stated). The Wigner–Seitz radius r s is set equal to 4 a 0 corresponding to the Na metal, which is a prototype system for the jellium description. Each nanoparticle has a closed shell structure and consists of N e =1,074 electrons. The cluster radius is r s =40.96 a 0 ( 2.17 nm), and the Fermi energy of the system is at 2.9 eV below the vacuum level. The time-dependent electron density is given by with the summation running over all occupied (occ) KS orbitals ψ j ( r , t ). The time evolution of KS orbitals is given by the time-dependent Scrödinger equation where the external laser radiation is treated in the velocity gauge: Here, is the kinetic energy operator, with being the vector potential of the laser field. We assume that the external radiation is polarized along the z -direction, that is, along the symmetry axis of the dimer. We use the non-retarded approximation, which is fully justified because of the small size of the system. The effective KS potential V eff ( r , t ) is then obtained as: where the first term is the Hartree potential V H and the second term is the exchange correlation potential. The switching function of the positive background density ( R cl − r ) varies smoothly from 0 to a constant value 1 at the cluster boundary over a short length scale of δ =0.2 a 0 . It is normalized in such a way so that the charge neutrality of the system is preserved. The smooth termination profile and, most importantly, the spill-out of the electron density outside the cluster [46] , [47] result in a dipolar plasmon appearing at ω pl =2.98 eV, which is somewhat lower than the classical value , consistent with the results from the literature. The linear properties of the system are obtained from the response to a weak impulsive potential in the absence of the external laser field ( ). To this end, the V eff has been set as: V eff = V H + V xc + ξδ ( t ), where ξ is a small constant ( ξ =0.003 eV). The Fourier time-to-frequency transform of the near-fields and the induced dipole moment allows the calculation of the frequency-resolved field enhancement as well as the optical absorption cross-section given by σ abs =(4 πω / c )Im{α( ω )} with α ( ω ) being the dipolar polarizability of the system. We have also calculated the induced fields and currents through the junction by applying an external 20-fs laser pulse with gaussian spectral profile centered at the frequency of interest. Both (impulsive potential and external laser pulse) methods yield consistent results. For the small dimer in Fig. 3 , the absorption and extinction cross-section can be considered to be equal. The numerical procedure to solve equation (6) is similar to the one used in the one-electron wave packet propagation, and it is detailed elsewhere [48] , [49] , [50] , [51] . The initial conditions ψ j ( r , t =0) correspond to non-perturbed K–S orbitals of the ground-state system. To avoid complications linked with the change of the number of electrons in the computation box, we have not introduced the complex absorbing potentials [52] at the boundaries of the mesh. Indeed, for the linear response calculations and at low laser intensities no noticeable ionization occurs. Tunnelling probability In the case of two small spheres forming a dimer, the surface curvature may have a role. However, to keep the consistency of the approach and to test the applicability in this (extreme) situation, we have described the conductivity of the junction within the planar surface approximation in equation (5). The transmission probability T (Ω, l ) was calculated using the effective one-electron potentials extracted from the density functional studies of the nanosphere dimer with separation distance D = l , that is, l corresponds to the separation between the closest points of the spheres measured from the jellium edges. This choice guarantees that along the interparticle axis z , where the tunnelling current is the strongest, the QCM calculations rely on the same tunnelling probability as the one implicitly present in the TDDFT calculation, thus allowing for a direct and exact comparison of both methods (QCM and QM within TDDFT). In the case of large gold particles, we use the jellium description of gold based on the model potentials developed earlier [53] in the simpler flat-plane junction, and account for the long-range image-potential interactions in the gold–gold junction [28] . Parametrization in the QCM The validity of the parameterization used to describe the tunnelling damping γ g ( l ) can be tested from a microscopic analysis of the amplitude and phase of the tunnelling current in the quantum-mechanical TDDFT calculations where an external laser pulse illuminates a small metallic dimer. In this approach, which, in contrast to the SSTM case, can be applied to arbitrarily small separations, the current is calculated directly from the wavefunctions of the electrons. A very good agreement between the full TDDFT calculations and our exponential parametrization used in the QCM is obtained both for the phase and amplitude of the resistive conductivity (explicit comparison shown in Supplementary Fig. S2 ). Integration of the QCM in classical calculations To calculate the optical response of a system within the QCM, we need to describe the plasmonic cavity by means of a local dielectric function ( ω ) that incorporates the elements of the quantum-mechanical electron tunnelling between the nanoparticles. The dependence of the local dielectric function ( l , ω ) on the separation distance l for each point in the transverse plane of the gap ( x , y ) results in an inhomogeneous junction where the local dielectric permittivity depends on its distance from the symmetry axis ( ( l ( x , y ), ω )). The QCM thus requires to solve Maxwell's equations in an inhomogeneous system. We use the standard boundary element method [27] as the classical solver, but the QCM can be equally well integrated in any other numerical solver of Maxwell's equations. A sufficiently fine grid was used that all the results are fully converged. Following an approach analogous to the Derjaguin approximation [54] , [55] , to solve the classical response in the inhomogeneous system within the boundary element method, we divide the gap into a sufficient number n of cylindrical shells, as schematically illustrated in Fig. 2b , with each i th shell characterized by a dielectric permittivity i = ( li , ω ) where l i is the corresponding longitudinal length of the i th shell. In our calculations, results were converged typically with use of only eight of such shells. This description thus assumes that the key parameters to describe the fictitious material are the separation distance l i at a given point ( x i , y i ) of the gap and the properties of the tunnelling at that particular point determined by the transmission probability T i and the local damping γ i . Any other dependence on the local shape of the object is neglected. To implement the solution of Maxwell's equations in large metallic systems forming a gap, the materials outside the gap are characterized by a classical dielectric function 0 =1 for the surrounding vacuum and by a homogeneous and isotropic local dielectric function m given by the Drude model with plasma frequency ω p and damping γ p to describe the metal in the particles, as depicted in Fig. 2b . When solving the Maxwell's equations to obtain the electrodynamical response of the full plasmonic system, the separation between the bulk metals and the surrounding media is assumed to be sharp, and a standard local classical description is adopted to describe the dielectric properties outside the gap within the QCM approach. Nevertheless, a non-local approach [14] is also fully compatible with the QCM presented here and could be implemented straightforwardly. However, for large plasmonic systems and narrow junctions, quantum-mechanical electron tunnelling is the major non-local effect that determines the optical response of the system, dominating over other non-local effects arising from the spill-out of electrons from regions outside the gap that might produce slight corrections. We note that the results from the QCM calculations agree very well with the results from the QM approach, which fully accounts both for non-locality induced by spill-out and by electron tunnelling, and charge transfer effects in the system. How to cite this article: Esteban R. et al . Bridging quantum and classical plasmonics with a quantum-corrected model. Nat. Commun. 3:825 doi: 10.1038/ncomms1806 (2012).